High performance piezoelectric devices based on aligned arrays of nanofibers of poly(vinylidenefluoride-co-trifluoroethylene) Multifunctional capability, flexible design, rugged lightweight construction and self-powered operation are desired attributes for electronics that directly interface with the human body or with advanced robotic systems. For these applications, piezoelectric materials, in forms that offer the ability to bend and stretch, are attractive for pressure/force sensors and mechanical energy harvesters. Here, we introduce a large area, flexible piezoelectric material that consists of sheets of electrospun fibres of the polymer poly[(vinylidenefluoride- co -trifluoroethylene]. The flow and mechanical conditions associated with the spinning process yield free-standing, three-dimensional architectures of aligned arrangements of such fibres, in which the polymer chains adopt strongly preferential orientations. The resulting material offers exceptional piezoelectric characteristics, to enable ultra-high sensitivity for measuring pressure, even at exceptionally small values (0.1 Pa). Quantitative analysis provides detailed insights into the pressure sensing mechanisms, and establishes engineering design rules. Potential applications range from self-powered micro-mechanical elements, to self-balancing robots and sensitive impact detectors. An emerging development trajectory in electronics focuses on portable and flexible devices for applications such as those that involve integration with the human body, as health/wellness monitors, surgical tools, sensor networks, artificial muscles and engineered tissue constructs [1] , [2] , [3] , [4] . In the field of robotics, similar technologies can be important in efforts to optimize human-like manipulation schemes for robust modes of interaction in complex daily environments, at home or at work [5] . Flexible, rugged and lightweight construction are key requirements, for both areas. Devices that exploit mechanical motions as natural sources of power can be particularly valuable [6] , [7] , [8] , [9] , [10] . Likewise, precision tactile sensors might represent first steps toward realization of artificial, electronic skins that mimic the full, multi-modal characteristics and physical properties of natural dermal tissues, for potential uses in robotics and human healthcare alike. Advanced materials will be critical to progress, particularly for integrated arrays that offer high sensitivity in the low-pressure regime (<1 kPa). Previous examples include flexible, matrix-type arrays of pressure or strain sensors based on conductive rubbers [11] , [12] , [13] . Although such sensors have simple designs, their performance is modest, with pressure sensitivities around 0.5 kPa ( [11] ) and response slopes, in terms of percentage changes in resistivity with pressure, of 0.05% (kPa) −1 ( [12] ). Recent component level studies indicate that sensitivities as high as 0.4 Pa ( [14] ) and 3 Pa ( [15] ) can be achieved with triboelectric sensors and with air-gap capacitors, respectively. These systems are of interest for many uses, but they suffer from undesirable sensitivities to static electricity, stray capacitances and temperature changes. Piezoelectric polymers are especially promising for devices with this type of functionality, because they can exploit deformations induced by small forces, through pressure, mechanical vibration, elongation/compression, bending or twisting [16] . These materials combine structural flexibility, ease of processing and good chemical resistance, with large sensitive areas, simplicity in device design and associated potential for low cost implementation. Current state-of-the-art pressure sensors based on piezoelectric polymers mainly rely on thin film geometries. In parallel plate configurations [17] , or combined with transistors on polymide substrates, such films enable precise pressure sensing, at a level suitable for detecting the touch of a finger (~2 kPa) [18] . Poly(vinylidenefluoride) (PVDF) and its copolymers have particularly attractive piezoelectric properties in these geometries. Their plastic behaviour makes them suitable for high-throughput processing [16] , [19] based on moudling, casting, drawing and spinning. Their carbon-fluorine chemistry renders them highly resistant to solvents, acids and bases. A disadvantage is that achieving good performance (~kPa sensitivity) requires electrical poling to create maximum polarization in the direction orthogonal to the film plane [20] , [21] . This process constrains engineering design options and, at the same time, requires multiple preparatory steps. Emerging techniques in nanofabrication have the potential to optimize piezoelectric responses, expand the range of device structures that can be considered and simplify processing. For example, near and far field electrospinning methods can produce piezoelectric nanofibers, in which the associated extensional forces and electric fields naturally cause local poling and, by consequence, enhanced properties. Previous reports, however, describe fibres of this type only in the form of non-woven mats or isolated strands [22] , [23] , [24] , [25] , [26] . In particular, previously reported arrays of fibres of PVDF are present as monolayers or few layer coatings, with modest degrees of alignment (±20°) and separations of a few microns [24] . Furthermore, these fibres require high-electric fields for poling, provided by either post-processing [24] or near-field electrospinning [25] . Under comparable bending conditions, the current outputs of devices produced with such fibres are <5 nA and the voltages are in the range of 1–20 mV ( [24] , [25] ). Realistic device functionality under various stress conditions, such as compression and bending, can be best achieved with high volumetric densities of aligned arrays of fibres. These high densities are difficult to obtain by means of gap collectors or near-field spinning. Gap collectors generally have poor capabilities in producing large area samples [27] with high degrees of alignment and uniformity in coverage because of the critical dependence on residual charges on the fibres in the gap. On the other hand, near-field methods typically involve direct serial writing, which is unsuitable for realizing large area and multilayered aligned arrays of fibres. Here, we describe procedures that allow this type of architecture, and demonstrate the key features using free-standing, high-density arrays as a piezoelectric textile that can cover large areas (tens of cm 2 ). The resulting materials are mechanically robust and can be handled easily, with the capability to be bent or twisted without fracture. Under bending conditions, these fibres exhibit currents up to 40 nA and voltage about 1.5 V. Furthermore, detailed characterization and modelling studies indicate distinctive piezoelectric features, owing to underlying alignment at the scale of both the polymer chains and the fibres. Flexible pressure sensors built simply by establishing electrical contacts to the ends of the aligned fibres show excellent sensitivity in the low-pressure regime (0.1 Pa) and respond to both compressive and bending forces. Alternative device architectures allow other modes of use, in sensors of acceleration, vibration and orientation. Free-standing arrays of aligned nanofibers The optimal fibre spinning process occurs with a potential of 30 kV between a nozzle tip with inner diameter of 200 μm, fed by a syringe pump at a flow-rate of 1 ml h −1 , and a collector at a distance of 6 cm. See Fig. 1 . A unique feature of this setup is a collector disk with sub-cm width that rotates at angular speeds as high as 4,000 r.p.m., corresponding to linear speeds>16 m s −1 at the collector surface. The consequence of this arrangement is that it forces overlapping fibres, which yields mesoscopic joints and significantly enhanced mechanical robustness. Using a high boiling point (that is, slowly evaporating) solvent such as DMF (Tb: 154 °C) helps to ensure the formation of such joints as shown in Fig. 2 . Joint lengths range from hundreds of nanometres to tens of micrometres. In most of cases, fibres are arranged in groups where mutual adhesion through formation of these joints takes place ( Fig. 2a ). Occasionally, joined fibres remain strictly parallel, twist or cross at certain angles with respect to each other ( Fig. 2c–e ). The present set-up enables fibre arrays with widths of 0.8 cm, lengths of 25 cm and thicknesses of 10–40 μm, depending on the spinning time duration ( Fig. 1b ). The average fibre diameter for materials studied here is 260 nm, with a distribution that appears in Fig. 1d . The arrays have densities of ~2 × 10 7 fibres per mm 2 of cross-sectional area, and an overall porosity of 65%. The alignment is uniform over many centimeters ( Fig. 1e and Supplementary Fig. S1 ). Fast Fourier transforms (FFTs) [28] of scanning electron micrographs yield quantitative information on the degree of alignment, as shown in Fig. 1f . In the following, conventional, randomly oriented fibre mats, produced by spinning onto a static collector, and spin-cast thin films provide points of comparison. 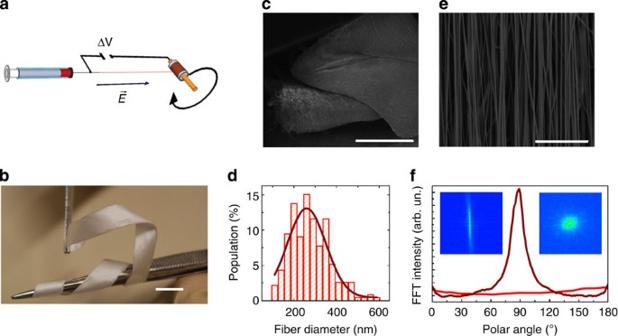Figure 1: Arrays of highly aligned piezoelectric nanofibers of poly[(vinylidenefluoride-co-trifluoroethylene]. (a) Schematic illustration of the experimental setup for electrospinning highly aligned arrays of oriented nanofibers of aligned polymer chains of poly[(vinylidenefluoride-co-trifluoroethylene].indicates the direction of the electric field and ΔV is the applied bias. (b) Photograph of a free-standing film of highly aligned piezoelectric fibres. Scale bar, 1 cm. (c) SEM micrograph of fibre arrays intentionally folded many times to highlight flexibility and mechanical robustness (scale bar, 400 μm). (d) Typical fibre diameter distribution and fit by a Gaussian curve (solid line). (e) SEM micrograph of fibre arrays (scale bar, 10 μm). (f) Radial intensity distribution versus detection angle (0–180°) for aligned arrays (wine line peak) and random mats (red line at bottom) of fibres. Insets: two-dimensional FFT images generated from aligned (left inset) and randomly oriented (right inset) fibres. In random mats, a highly symmetric, circular distribution of the pixel intensity confirms the un-oriented arrangement of fibres and correspondingly, a featureless behaviour of the radial pixel intensity versus angle. This distribution in fact, indicates that the frequency at which specific pixel intensities occurs in the corresponding data image is identical in any direction and no peaks can be appreciated by plotting the sum of the pixel intensity as a function of the degree in the interval 0°–360°. On the contrary, aligned fibres generate a highly anisotropic, elliptical two-dimensional FFT profile with the major axis oriented parallel to alignment axis. Full-width at half maximum of the radial intensity distribution=16°. Figure 1: Arrays of highly aligned piezoelectric nanofibers of poly[(vinylidenefluoride- co -trifluoroethylene]. ( a ) Schematic illustration of the experimental setup for electrospinning highly aligned arrays of oriented nanofibers of aligned polymer chains of poly[(vinylidenefluoride- co -trifluoroethylene]. indicates the direction of the electric field and ΔV is the applied bias. ( b ) Photograph of a free-standing film of highly aligned piezoelectric fibres. Scale bar, 1 cm. ( c ) SEM micrograph of fibre arrays intentionally folded many times to highlight flexibility and mechanical robustness (scale bar, 400 μm). ( d ) Typical fibre diameter distribution and fit by a Gaussian curve (solid line). ( e ) SEM micrograph of fibre arrays (scale bar, 10 μm). ( f ) Radial intensity distribution versus detection angle (0–180°) for aligned arrays (wine line peak) and random mats (red line at bottom) of fibres. Insets: two-dimensional FFT images generated from aligned (left inset) and randomly oriented (right inset) fibres. In random mats, a highly symmetric, circular distribution of the pixel intensity confirms the un-oriented arrangement of fibres and correspondingly, a featureless behaviour of the radial pixel intensity versus angle. This distribution in fact, indicates that the frequency at which specific pixel intensities occurs in the corresponding data image is identical in any direction and no peaks can be appreciated by plotting the sum of the pixel intensity as a function of the degree in the interval 0°–360°. On the contrary, aligned fibres generate a highly anisotropic, elliptical two-dimensional FFT profile with the major axis oriented parallel to alignment axis. Full-width at half maximum of the radial intensity distribution=16°. 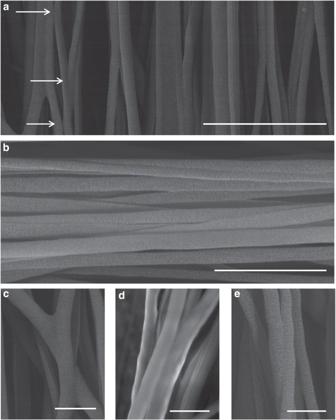Figure 2: Mesoscopic inter-fiber joints. (a) SEM micrographs of fibres highlighting points of merging (joints) between two or more adjacent fibres and (b) their typical arrangement in groups where strong merging takes place (arrows indicate examples of joints in the micrographs. Scale bars, 3 and 2 μm, respectively). Magnification of crossed (c; scale bar, 1 μm), adjacent (d; scale bar, 1 μm) and twisted (e; scale bar, 500 nm) fibre geometries at the joints. Full size image Figure 2: Mesoscopic inter-fiber joints. ( a ) SEM micrographs of fibres highlighting points of merging (joints) between two or more adjacent fibres and ( b ) their typical arrangement in groups where strong merging takes place (arrows indicate examples of joints in the micrographs. Scale bars, 3 and 2 μm, respectively). Magnification of crossed ( c ; scale bar, 1 μm), adjacent ( d ; scale bar, 1 μm) and twisted ( e ; scale bar, 500 nm) fibre geometries at the joints. Full size image X-ray photoelectron spectroscopy (XPS) indicates a ratio of co-polymer poly[(vinylidenefluoride- co -trifluoroethylene] [P(VDF-TrFe)] of 0.73:0.27, in agreement with the ratio before electrospinning ( Supplementary Fig. S2 and Supplementary Note 1 ). P(VDF-TrFe) generally exhibits good piezo- and ferro-electric behaviour and a single all-trans polar crystalline phase (β-phase) that is stable at room temperature [29] . The ferroelectricity stems from electrical dipoles created by hydrogen and fluorine atoms in the VDF molecules, which are positioned perpendicularly to the polymer backbone [30] . X-ray diffraction (XRD) patterns provide information on the long-range order and the crystal structure of both aligned arrays and random networks ( Fig. 3a ). The results indicate that the overall crystallinity of the material in the aligned arrays is ~48%, while that for the random mats is 40%. The former value is, in fact, comparable to that of the best previous results produced in thin films by stretching [31] . A distinguishing feature of the fibre arrays is that the rotating collector significantly enhances the fraction of the polar β-phase, as is shown in the X-ray results of Fig. 3a and in the polarized Fourier transform infrared (FTIR) spectra of Fig. 3c . The polar β-phase bands [32] , [33] , [34] appear distinctly at 508, 846, 1285 and 1431, cm −1 . By contrast, the bands of the non-polar α-phase (532, 612, 765, 796, 854, 870, 970 cm −1 ) are not appreciable. The fraction of β-phase determined by analysis of these FTIR results [31] is close to 85%. Furthermore, the spectra show a significant increase in the intensity of bands associated with vibrations that depend on chain orientation (1,076 and 1,400 cm −1 ) [35] for light polarized along the longitudinal axis of the fibre (blue line in Fig. 3d ), and a corresponding reduction in the intensity of bands sensitive to dipolar orientation (508, 846, 1,285 and 1,431 cm −1 ). These results suggest a preferential alignment of the main molecular chains along the fibre longitudinal axis and, at the same time, an enhancement of the orientation of piezoelectric active dipoles (C-F) in the direction perpendicular to this axis ( Supplementary Fig. S3a ). This finding is consistent with a preferential dipolar alignment along the direction of the electrospinning field during fibre collection ( Fig. 1a ). FTIR spectra collected under different polarization conditions highlight an exceptional level of alignment, even compared with previous experiments using rotating collectors [26] , for which the fibres exist in moderately aligned mats. For instance, the ratio of intensities of absorption bands at 846 and 1285, cm −1 ( [35] ), which are indicative of the symmetric stretching vibration of the piezoactive (C-F) dipoles, under different polarizations are 2 and 2.6, respectively, about two times higher than corresponding ratios in previous reports [26] . This result is attributable to the combined effects of four-fold higher rotational speed (namely, 2.3-times higher linear speed) of our collector, which causes tighter mutual alignment of nanofibers and concomitantly stronger stretching, and to excellent fibre alignment. We note that such polarization effects are not observed in free-standing P(VDF-TrFe) films ( Supplementary Fig. S3c ), where preferential chain alignment is not expected, or in random mats, mainly because of the random alignment of fibres ( Supplementary Fig. S3d ) (We note that the mats showed higher degree of crystallinity compared with the films (40% versus 35%), consistent with expected effects of electrospinning.) 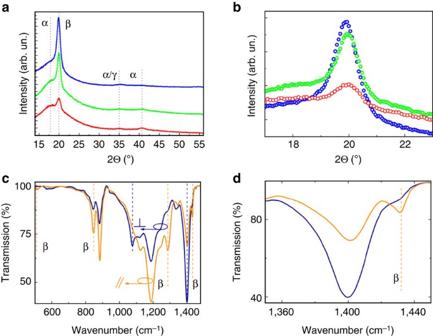Figure 3: Characterization of morphologies and properties of arrays. (a) XRD patterns (Cu radiation with wavelength=0.15418, nm) from aligned fibres (top blue line), randomly oriented fibres (middle green line) and a film (bottom red line) collected with the fibres length oriented parallel to the diffraction plane (azimuthal rotationф=0). The patterns are vertically shifted to facilitate comparison with the results. (b) Magnified view of XRD spectra at 2θ20°, which corresponds to diffraction in (110) plane and represents the β-phase. Although the peak is visible in all samples (aligned arrays of fibres (blue dots), random mats of fibres (green dots) and bare films (red dots), it is dominant in the aligned nanofibers arrays, where the contribution from the α-phase is insignificant. (c) FTIR spectra measured under different incident beam polarizations for aligned fibers. Light is polarized parallel (orange line) and perpendicular (blue line) to the direction of the electric field used in electrospinning. Similar spectra were measured at different values of the electric field. (d) Magnified view of the low energy region of the FTIR spectra, highlighting the increase of the intensity of transitions sensitive to chain orientation (1,400 cm−1) for light polarized along the axis of the fibres (blue line). Figure 3: Characterization of morphologies and properties of arrays. ( a ) XRD patterns (Cu radiation with wavelength=0.15418, nm) from aligned fibres (top blue line), randomly oriented fibres (middle green line) and a film (bottom red line) collected with the fibres length oriented parallel to the diffraction plane (azimuthal rotation ф =0). The patterns are vertically shifted to facilitate comparison with the results. ( b ) Magnified view of XRD spectra at 2 θ 20°, which corresponds to diffraction in (110) plane and represents the β-phase. Although the peak is visible in all samples (aligned arrays of fibres (blue dots), random mats of fibres (green dots) and bare films (red dots), it is dominant in the aligned nanofibers arrays, where the contribution from the α-phase is insignificant. ( c ) FTIR spectra measured under different incident beam polarizations for aligned fibers. Light is polarized parallel (orange line) and perpendicular (blue line) to the direction of the electric field used in electrospinning. Similar spectra were measured at different values of the electric field. ( d ) Magnified view of the low energy region of the FTIR spectra, highlighting the increase of the intensity of transitions sensitive to chain orientation (1,400 cm −1 ) for light polarized along the axis of the fibres (blue line). Full size image Experimental and theoretical studies of piezoelectric sensor These characteristics make fibre arrays promising as building blocks for ultrasensitive piezoelectric sensors. Devices, formed simply by establishing electrical contacts to the ends of a ribbon-shaped sample of fibre arrays on a flexible polyimide (PI) support (Kapton; thickness selected between 75 and 225 μm), reveal large response to even minute applied pressures ( Fig. 4 ). To evaluate the sensitivity quantitatively, a soft elastomer (PDMS posts in Fig. 4a ) delivered well-defined levels of pressure to the arrays, while the electrical response was measured. Data in Fig. 4c highlight well-behaved, linear variations in the output voltage with pressure, for various values of the effective contact areas between 9 and 36 mm 2 (squares with sides L eff ; Fig. 4b ), with slopes between 0.41 and 0.79 mV Pa −1 . At ranges of pressure between 0.4 and 2 kPa, the devices show further improved sensitivity, that is, 1.1 V kPa −1 . For a given pressure (10 Pa, L eff =3 mm), the output voltage does not change significantly with length of the fibre array, over a range between 2 and 8 cm). Even without sensitive voltmeters, this level of response enables accurate measurement of compressive pressures as small as 0.1 Pa ( Fig. 4d ). These response slopes, which provide a measure of sensitivity that is independent of data acquisition systems, together with the observed broad dynamic range, provide unique operation compared with that provided by other sensors based on capacitive (0.55 kPa −1 in units of relative capacitance, in a range of 0.5–2 kPa) [15] and piezoelectric (0.1 mV Pa −1 , in a range of 0.01–30 Pa) [18] effects, as well as most force and tactile sensing methods that are currently available for in-hand manipulation in robotics [36] . 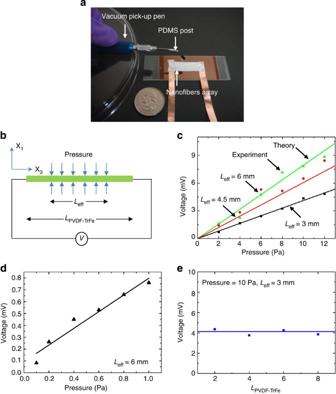Figure 4: Experimental and theoretical studies of responses of pressure sensors. (a) Photograph of the manipulator used to apply pressures, for the purpose of studying the voltage response. (b) Schematic illustration of an analytical model for the response of arrays of P(VDF-TrFe) fibres under applied compression −palongx1direction over the effective contact length (Leff).LPVDF-TrFeis the total length of the P(VDF-TrFe) fibre array. (c) Experimental (symbols) and theoretical (lines) pressure response curves at differentLeff. (d) Experimental (symbols) pressure response curve in the low-pressure regime (0.1–1 Pa) atLeff=6 mm. The line corresponds to a linear fit. (e) Experimental (symbols) and theoretical (lines) response at differentLPVDF-TrFe(applied pressure=10 Pa,Leff=3 mm). Figure 4: Experimental and theoretical studies of responses of pressure sensors. ( a ) Photograph of the manipulator used to apply pressures, for the purpose of studying the voltage response. ( b ) Schematic illustration of an analytical model for the response of arrays of P(VDF-TrFe) fibres under applied compression − p along x 1 direction over the effective contact length ( L eff ). L PVDF-TrFe is the total length of the P(VDF-TrFe) fibre array. ( c ) Experimental (symbols) and theoretical (lines) pressure response curves at different L eff . ( d ) Experimental (symbols) pressure response curve in the low-pressure regime (0.1–1 Pa) at L eff =6 mm. The line corresponds to a linear fit. ( e ) Experimental (symbols) and theoretical (lines) response at different L PVDF-TrFe (applied pressure=10 Pa, L eff =3 mm). Full size image The observed behaviours can be well explained by an analytic piezoelectric model. Consider a resultant projected component of piezoactive dipoles along the longitudinal axis of the fibres, x 3, as induced by the deformation ( Fig. 4b ). The fibre array are transversely isotropic with elastic, piezoelectric, and dielectric constants c ij , e ij , and k ij ( [37] ), respectively. For an applied compression - p along the x 1 direction (normal to fibres, Fig. 4a ) over an effective contact length L eff ( Fig. 4a ), the strain ε 11 and electric field E 3 along the poling direction are obtained from the constitutive relation − p = c 11 ε 11 − e 31 E 3 and D 3 = e 31 ε 11 + k 33 E 3 (see Supplementary Note 2 for details), where D 3 is the electric displacement along the poling direction. When the fibre arrays are connected to a voltmeter, E 3 and D 3 are related to the measured voltage V and current I by V = L eff E 3 and , where h PVDF-TrFe =20 μm and w PVDF-TrFe =8 mm are the thickness and width of the fibre array cross section, respectively. The voltage and current are then related by the resistance of the voltmeter, such that the voltage across L eff (see Supplementary Note 2 for details) is where and . For , Equation (1) agrees well with the experimental results shown in Fig. 4b for a wide range of pressures p and the three effective contact lengths L eff =3, 4.5 and 6 mm used in the experiments. The value of reaches or exceeds those achieved in films with extreme stretching and poling (for example, ~0.045–0.094 Vm N −1 ( [38] )). Equation (1) also suggests that the voltage is independent of the total length L PVDF-TrFe ( Fig. 4e ) of the P(VDF-TrFe) fibre arrays, which is also consistent with experimental results of Fig. 4c . Additional behaviours were observed in dynamic bending experiments performed using fibre arrays on PI films with thicknesses between 75 and 225 μm. A flexural endurance tester (IPC, CK-700FET) subjected the samples to cycling bending tests at 1 Hz ( Fig. 5c ) and 2 Hz ( Fig. 5d ). During compression, the sample buckled to generate a bent shape ( Fig. 5a ), with curvature consistent with simple mechanics considerations. The measurements showed a periodic alternation of positive and negative output peaks, corresponding to the application and release of the buckling stress, respectively, ( Fig. 5b ). The ranges of short-circuit current and voltage outputs were 6–40 nA and 0.5–1.5 V, respectively. Both responses increased with increasing PI thickness and with increasing bending frequency. The maximum current (40 nA) and voltage (1.5 V) were observed from fibre arrays on 225 μm thick PI substrates at 2 Hz. Tests of up to 1,000 cycles of bending and relaxing revealed no significant changes in output voltage or current. 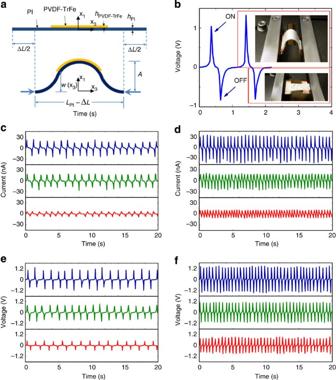Figure 5: Experimental and theoretical studies of responses of flexural sensors. (a) Schematic illustration of an analytical model for the coupling of mechanical deformation and piezoelectric response during bending.hPVDF-TrFeandhPIare the thicknesses of the P(VDF-TrFe) fibre array and of the PI substrate, respectively.LPIis the length of the PI substrate. Under compression, the PI substrate buckles into a sinusoidal form represented by the out-of-plane displacementwand the amplitudeA,which is related to compression ΔLof the substrate. (b) Measured voltage response of an array of P(VDF-TrFe) fibres under cycling bending at 1 Hz. The top and bottom insets show photographs of the device during bending and release, respectively. (c,d) Measured short- circuit output current and (e,f) voltage under dynamic bending tests at 1 Hz (left panels;c,e) and 2 Hz (right panels;d,f). Experiments used devices onto PI substrates with different thickness. From bottom to top, the PI thicknesses are 75 μm (red line), 150 μm (green line), 225 μm (blue line). Figure 5: Experimental and theoretical studies of responses of flexural sensors. ( a ) Schematic illustration of an analytical model for the coupling of mechanical deformation and piezoelectric response during bending. h PVDF-TrFe and h PI are the thicknesses of the P(VDF-TrFe) fibre array and of the PI substrate, respectively. L PI is the length of the PI substrate. Under compression, the PI substrate buckles into a sinusoidal form represented by the out-of-plane displacement w and the amplitude A, which is related to compression Δ L of the substrate. ( b ) Measured voltage response of an array of P(VDF-TrFe) fibres under cycling bending at 1 Hz. The top and bottom insets show photographs of the device during bending and release, respectively. ( c , d ) Measured short- circuit output current and ( e , f ) voltage under dynamic bending tests at 1 Hz (left panels; c , e ) and 2 Hz (right panels; d , f ). Experiments used devices onto PI substrates with different thickness. From bottom to top, the PI thicknesses are 75 μm (red line), 150 μm (green line), 225 μm (blue line). Full size image As with applied pressure, simple analytical models can account for the behaviours under bending(see Supplementary Note 3 for details). Under compression the PI substrate of length L PI buckles into a sinusoidal form represented by the out-of-plane displacement , where the origin of coordinate x 3 is at the center of the substrate, and the amplitude A is related to compression Δ L of the substrate by ( [39] ). Here, the critical compression to trigger buckling, ~1 μm for 150 μm-thick and 6 cm-long PI substrate, is negligible as compared with Δ L =3 cm in the experiments. The strain along the poling direction x 3 at the mid-plane of the fibre arrays is given by , where h PI and h PVDF-TrFe are the thicknesses of PI substrate and P(VDF-TrFe) fibre arrays, respectively. Its strain ε 11 along x 1 and electric field E 3 along the poling direction are obtained from the constitutive relation 0= c 11 ε 11 + c 13 ε 33 − e 31 E 3 and D 3 = e 31 ε 11 + e 33 ε 33 + k 33 E 3 , where D 3 is the electric displacement along the poling direction, and is a constant to be determined. For short-circuit current measurement between two ends of the P(VDF-TrFe) fibre arrays, the voltage across the length of P(VDF-TrFe) L PVDF-TrFe is zero, which, together with the above equations, gives , where is the effective piezoelectric constant. The current I is then obtained from , where w PVDF-TrFe is the width of P(VDF-TrFe) fibre arrays (such that h PVDF-TrFe w PVDF-TrFe is the cross section area). For a representative compression with the maximum compression and period t 0 =0.5 and 1 s as in experiments, the maximum current is given by For L PVDF-TrFe =2.5 cm and three thicknesses of PI substrate h PI =75, 150 and 225 μm as in experiments, Equation (2) gives the range of I max ~14–27 nA for t 0 =0.5 s and 5.6–14 nA for t 0 =1 s, while experiments give 10–33 nA and 6.5–26 nA for t 0 =0.5 and 1 s, respectively. Here, the effective piezoelectric constant for the fibre arrays is taken as , which is larger than that for films (~−0.4 C m −2 ) [37] because of the strong anisotropy of arrays due to their fibrous structure. For voltages measurements, V is no longer zero. The electric displacement becomes . The current is also related to the voltage V and the resistance R of the voltmeter by I = V / R , which gives , or equivalently For and the initial condition V ( t =0)=0, the maximum voltage is given by For three thicknesses of PI substrate h PI =75, 150 and 225 μm as in experiments and a resistance of the voltmeter R =70 MΩ, consistent with values resulting from independent resistance measurements, equation (4) gives a range of V max 0.81–2.1 V for T =0.5 s and 0.29–0.85 V for t 0 =1 s, while experiments give 0.79–1.3 V and 0.49–1.0 V for t 0 =0.5 and 1 s, respectively. Pyroelectric response The pyroelectric response in these systems was also studied by measuring the current and voltage output upon heating/cooling cycles with a temperature range of 6 K around room temperature ( Supplementary Fig. S4 and Supplementary Note 4 ) [40] , [41] , [42] . The measured pyroelectric coefficient [41] for the fibre arrays was ( Supplementary Fig. S5 ). For a constant heating/cooling rate 2.5 K min −1 ( Supplementary Fig. S6 ), the maximum voltage measured from the voltmeter was 1.9 μV when the fibre arrays were in contact with the top of the heater ( Supplementary Fig. S4b ). The maximum voltage obtained from an analytic pyroelectric model is which was also given by Lubormisky et al . [41] , and is also shown in Supplementary Note 5 . Equation (5) gives 1.81 μV for dT/dt =2.5 K min −1 and α , R , h PVDF-TrFe and w PVDF-TrFe in the experiments (see in Supplementary Note 5 for details). This value is in good agreement with the measured value, 1.9 μV. For the same set of parameters, Equation (5) indicates that, at heating rates of ~6.5 K min −1 , the pyroelectric voltage is only 5.6% of the piezoelectric voltage (0.084 mV) at the lower end of the range of pressure sensitivity (0.1 Pa, and L eff =6 mm in equation (1) for the type of tests reported here). We note, however, that for most envisioned applications such as measurements of sound waves, pressure waves in arteries, mechanical vibrations, disturbances associated with breathing, motion in limbs and so on the timescales for mechanically induced change are, in many cases, different than those associated with characteristic thermal processes. Furthermore, in bio-integrated applications, the operating temperature range is narrow (<3 K), and the extent of mechanical deformation (in many cases) is large. Such circumstances enable any necessary separation of mechanical and thermal signals by frequency filtering as part of backend data processing, with no change in the devices. Additional sensory applications As demonstrators, we built devices capable of measuring vibration/acceleration and orientation. For the first, the fibre array serves as a diaphragm across a hole opened in a underlying plastic film, sealed over the closed cavity of a transparent box ( Fig. 6a ). Through the plastic film, movements are transmitted from the box frame to the array, which then operates as a vibrating mass of ~3 mg. 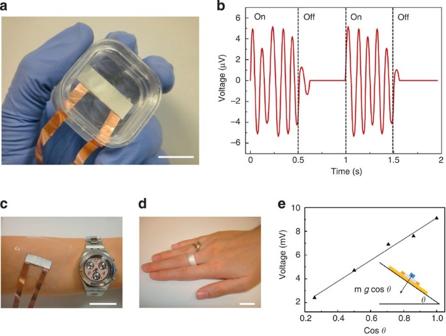Figure 6: Accelerometer and orientation sensor. (a) Photograph of a simple, P(VDF-TrFe) nanofiber-based accelerometer. Scale bar, 1 cm. (b) Output voltage collected from this device exposed to 70 dB sound intensity. (c,d) Photographs of a flexible device mounted on the skin of the arm and wrapped around a finger. Scale bar, 2 cm. (e) Characterization of an orientation sensor, based on a pressure sensor with an attached test mass. The output voltage changes with orientation angle,θ, in an expected manner. The inset provides a sketch of the device (yellow: PI; grey: fibres; blue: test mass) and the measurement geometry. Figure 6b displays the output voltage signal generated by this simple device, as response to environmental vibrations induced by sound pressure levels of 60–80 dB. The response included periodically alternating positive and negative voltage peaks, with a peak-to-peak output voltage that increases from 6–14 μV with sound intensity. These devices work in any orientation and can be mounted on any surface by means of transparent, skin-conformal plastic sheets ( Fig. 6c ). In a second example, a similar type of device, integrated on a solid support and with an attached test mass, acts as an orientation sensor. Measurements on a inclined plane with variable angle, as sketched in the inset of Fig. 6e , allow calibration of the response. Figure 6e shows the output voltage collected at different inclinations, which yields a response that is consistent with a gravitation constant, g =9.8 m s −2 [43] , measured with experimental uncertainties of a few per cent, mainly due to manual positioning of PDMS posts. Figure 6: Accelerometer and orientation sensor. ( a ) Photograph of a simple, P(VDF-TrFe) nanofiber-based accelerometer. Scale bar, 1 cm. ( b ) Output voltage collected from this device exposed to 70 dB sound intensity. ( c , d ) Photographs of a flexible device mounted on the skin of the arm and wrapped around a finger. Scale bar, 2 cm. ( e ) Characterization of an orientation sensor, based on a pressure sensor with an attached test mass. The output voltage changes with orientation angle, θ , in an expected manner. The inset provides a sketch of the device (yellow: PI; grey: fibres; blue: test mass) and the measurement geometry. Full size image Results presented here indicate that aligned P(VDF-TrFe) nanofibers can be formed into flexible, free-standing sheets, by use of electrospinning onto a fast rotating collector. The process yields alignment at both the level of the fibres and the polymers, thereby enabling excellent response and high piezoactive β-fraction without further processing (for example, electrical poling). Combining experimental and theoretical approaches, both details of the material and device performances are presented under different operating conditions. Simple pressure sensors exhibit excellent response in the extremely small pressure regime. Other simple devices can be constructed easily, including accelerometers, vibrometers and orientational sensors. The collective results suggest utility in a variety of sensor- and energy harvesting components, with lightweight construction, attractive mechanical properties and potential for implementation over large areas at low cost, with application opportunities in human motion monitoring and robotics. Electrospinning and electron microscopy P(VDF-TrFe) (75/25 weight%, Solvay Solexis) was dissolved in 3:2 volume ratio of dimethylformamide/acetone (DMF/acetone, Sigma Aldrich) at a polymer/solvent concentration of 21% w/w. Electrospinning was performed by placing 0.4–0.9 ml of solution into a 1.0 ml plastic syringe tipped with a 27-gauge stainless steel needle. The positive lead from a high voltage supply (XRM30P, 82 Gamma High Voltage Research) connected to the metal needle, for application of bias values around 25 kV. The solution was injected into the needle at a constant rate of 1 ml h −1 with a syringe pump (33 Dual Syringe Pump, Harvard Apparatus). A static collector made of a metallic plate covered with an Al foil, or a cylindrical collector (diameter=8 cm, Linari Engineering S.r.l), was placed at a distance between 3 and 20 cm from the needle and biased at −6 kV for the fabrication of random and aligned mats, respectively. To investigate the nature and structure of mesoscopic joints, arrays of fibres were made using solutions of PVDF-TrFe in acetone, methylethylketone (MEK), tetrahydrofuran (THF) and DMF/acetone at volume ratios from 4:1 to 1:4. We found that joints form only when using DMF/acetone. Continuous, free-standing, high-dense arrays of fibres can be achieved for DMF/acetone volume ratios in the range from 1:2 to 3:2. At the lowest DMF content, needle clogging interrupts electrospinning and thus limits the density of the arrays to 1 × 10 3 fibres per mm. At highest DMF content, fibres are discontinuous due to the presence of beads and necks. Here, the degree of mutual alignment is also strongly reduced. Extensive electrospinning experiments were also performed with acetone, THF and MEK by varying the PVDF-TrFe/solvent concentration in the range 12–21% (w/w). The results, which appear in Supplementary Fig. S7 , suggest that use of DMF is critically important in the formation of continuous, smooth fibres at high densities and with mesoscopic joints at crossing points. For purposes of comparison, PVDF fibres formed with the same experimental conditions were examined, to compare the morphological, crystallographic and mechanical properties against those of PVDF-TrFe ( Supplementary Figs. S8 and S9 ). Films of P(VDF-TrFe) with thicknesses of 10–40 μm were deposited by spin-coating at 800 r.p.m.. All the fabrication steps were performed at room temperature with air humidity of about 40%. The morphological analysis was performed by scanning electron microscope (s.e.m.) with a Nova NanoSEM 450 system (FEI), using an acceleration voltage around 5 kV and an aperture size of 30 μm. For quantitative analysis of alignment, SEM micrographs were converted to 8-bit grayscale TIF files and then cropped to 880 × 880 pixels. ImageJ software (NIH, http://rsb.info.nih.gov/ij ) supported by an oval profile plug-in (authored by William O’Connell) was used for radial summation of pixel intensities. All FFT data were normalized to a baseline value, and FFT images were rotated by 90° for better visualization. X-ray and spectroscopic characterization XPS spectra of fibres were collected using a Kratos Axis ULTRA X-ray photoelectron spectrometer with monochromatic Al Kα-excitation, 120 W (12 kV, 10 mA). To reduce the effects of surface charging, the monochromatic source was operated at a bias voltage of 100 V. Data were collected using the low magnification (FOV1) lens setting with a 2-mm aperture (200 μm analysis area) and charge neutralizer settings of 2.1 A filament current, 2.1 V charge balance and 2 V filament bias. Survey spectra were collected at a pass energy of 160 eV and high resolution spectra were recorded using a pass energy of 40 eV. The data were fitted with Gaussian–Lorentzian line shapes. The binding energy scale was referenced to the aliphatic C 1s line at 285.0 eV. IR spectroscopy was performed with an FTIR spectrophotometer (Spectrum 116 100, Perkin-Elmer Inc.), equipped with an IR grid polarizer (Specac Limited, UK), consisting of 0.12 μm wide strips of aluminium. The 4 mm wide beam, incident orthogonally to the plane of the sample, was polarized alternatively parallel or orthogonal to the main axis of fibre alignment. FTIR measurements performed on different samples and on different points of the same sample yielded similar results. A PANalytical X’pert MRD system, with Cu k-alpha radiation (wavelength 0.15418, nm), crossed-slit collimator as primary optics, and secondary optics consisting of a parallel plate collimator, a flat graphite monochromator and a proportional detector, was used for XRD measurements. A detailed scheme of the XRD set-up we used is reported in Supplementary Fig. S10 . The crystallinity of the fibres was calculated from the area of the diffraction peaks (above the background) divided by the area of the whole diffraction curve. During X-ray analysis, samples were mounted on a low-background quartz holder. The instrument’s contribution to the background in the diffraction data was determined by separate measurements of the quartz holder without samples. Pressure sensor fabrication and characterization P(VDF-TrFe) aligned fibre arrays were placed on 75–150 and 225 μm thick kapton film, and electric connections were established with copper films (25 μm thick) and silver paint (Ted Pella Fast Dring Silver Paint, 160040-30). Open loop voltage measurements were performed by using a DAQ (SMU2055) USB multimeter (6.5 digit resolution, Agilent Technologies) with input resistance of R=70 MΩ. Short-circuits current measurements were performed with a Semiconductor Parameter Analyzer (4155C Agilent Technologies) that has 10 fA measurement resolution. Signals were not amplified before acquisition. Pressure tests were performed using PDMS posts with calibrated weights in the milligram range, formed by replica moudling against photolithographically defined templates. A Vacuum Pick-up Pen with Bent Metal Probe, 1′′ Long, 3/32′′ Cup diameter (Ted Pella, Inc., Vacuum Pickup System, 115 V) was used to place the PDMS on the fibre arrays from calibrated distance to apply desired pressures. Upon impact, the PDMS posts adhered conformably and instantaneously, resulting in registered voltage spikes from the fibre array, digitized at 50 samples per second by the measurement system. These procedures allowed application of controlled pressures, in the low-pressure regime (0.1–12 Pa) onto an active P(VDF-TrFe) fibre array area of 9–18 mm 2 . (Conventional load cells are difficult to implement for measurements in this range of pressures and areas). We performed control experiments indicating that no significant signal is observed without the fibres and that interchanging the connections reversed the polarity of the output ( Supplementary Fig. S11 ). All measurements were performed at 20 °C. Bending measurements Cycling tests and bending experiments were performed by using IPC Flexural Endurance Tester (Model: CK-700FET). The two edges of the sample were fixed within two sliding stripes. The buckling radius measured from the middle of PI substrate (max curvature) is 74 mm. Additional sensory measurements A Personal Daq/3000 Series 16-bit/1-MHz USB Data Acquisition System was used to collect voltage signals from P(VDF-TrFe) fibre-based accelerometer. Orientation measurements were performed by placing devices on horizontal surfaces configured at a range of inclined angles. These experiments uses a PDMS test mass of 43 mg with L eff =6 mm. Upon impact, the PDMS mass adhered to the fibres, resulting in voltage spikes from the device. Experimental data reported in Fig. 4c were used to determine pressure values for voltage measurements at each angle. How to cite this article: Persano, L. et al . High performance piezoelectric devices based on aligned arrays of nanofibers of poly[(vinylidenefluoride- co -trifluoroethylene]. Nat. Commun. 4:1633 doi: 10.1038/ncomms2639 (2013).